Functional mechanisms underlying pleiotropic risk alleles at the 19p13.1 breast–ovarian cancer susceptibility locus A locus at 19p13 is associated with breast cancer (BC) and ovarian cancer (OC) risk. Here we analyse 438 SNPs in this region in 46,451 BC and 15,438 OC cases, 15,252 BRCA1 mutation carriers and 73,444 controls and identify 13 candidate causal SNPs associated with serous OC ( P =9.2 × 10 −20 ), ER-negative BC ( P =1.1 × 10 −13 ), BRCA1 -associated BC ( P =7.7 × 10 −16 ) and triple negative BC ( P -diff=2 × 10 −5 ). Genotype-gene expression associations are identified for candidate target genes ANKLE1 ( P =2 × 10 −3 ) and ABHD8 ( P <2 × 10 −3 ). Chromosome conformation capture identifies interactions between four candidate SNPs and ABHD8 , and luciferase assays indicate six risk alleles increased transactivation of the ADHD8 promoter. Targeted deletion of a region containing risk SNP rs56069439 in a putative enhancer induces ANKLE1 downregulation; and mRNA stability assays indicate functional effects for an ANKLE1 3′-UTR SNP. Altogether, these data suggest that multiple SNPs at 19p13 regulate ABHD8 and perhaps ANKLE1 expression, and indicate common mechanisms underlying breast and ovarian cancer risk. Genome-wide association studies (GWAS) have identified more than 100 different genetic susceptibility regions for breast cancer (BC) [1] , [2] , [3] , [4] , [5] , [6] and 20 regions for epithelial ovarian cancer (EOC) [7] , [8] , [9] , [10] , [11] , [12] , [13] . A few of these regions, and in some cases the same genetic variants, are associated with risks of both cancers (pleiotropy), suggesting there may be underlying functional mechanisms and biological pathways common to different cancers. The TERT-CLPTM1L locus (5p15) is one such example in which the same variants are associated with risks of oestrogen receptor (ER)-negative BC, BC in BRCA1 mutation carriers and serous invasive OC [10] . Few studies have comprehensively described the functional mechanisms underlying common variant susceptibility loci [10] , [14] , [15] , [16] , [17] , [18] . More than 90% of risk alleles lie in non-protein-coding DNA and there is now unequivocal evidence that susceptibility regions are enriched for risk-associated single-nucleotide polymorphisms (SNPs) intersecting regulatory elements, such as transcriptional enhancers, predicted to control the expression of target genes in cis [19] , [20] , [21] . Establishing causality for risk SNPs is very challenging; of the thousands of risk associations identified by GWAS, functional validation of causal variants using genome editing has only been experimentally performed for two SNPs, one for prostate cancer [22] using the CAUSEL pipeline and the other for obesity [23] . Thus, there is a critical need to identify the causal risk SNP(s) and the overlapping regulatory element(s) and the target gene(s) regulated in an allele-specific manner. Breast and high-grade serous OC share common genetic and non-genetic risk factors, with mutations in BRCA1 and BRCA2 the most significant risk factors for both cancers, suggesting similar biological mechanisms drive breast and OC development. A region on chromosome 19p13.1 has previously been associated with susceptibility to BC and OC in the general population, and to modify the risks of BRCA1 -related BC and BRCA2 -related OC [9] , [24] , [25] , [26] , [27] . Initial studies indicated that the association signal was centred around the SNP rs8170 located in the BRCA1 -interacting gene BABAM1 (ref. 9 ), and subsequent studies have refined the subtype specific BC risks associated with these SNPs [24] , [25] , [26] , [28] . In the current study, we hypothesized that the same functional mechanism underlies the 19p13.1 risk association in both BC and OC. To evaluate this hypothesis we performed genetic fine mapping in BC and OC patients and in BRCA1 mutation carriers, and performed a wide range of functional assays in breast and ovarian tissues and in vitro models to identify the likely causal alleles, and target regulatory elements and susceptibility gene(s). Our data indicate that multiple SNPs are involved in the regulation of ABHD8 and perhaps ANKLE1 at this locus. 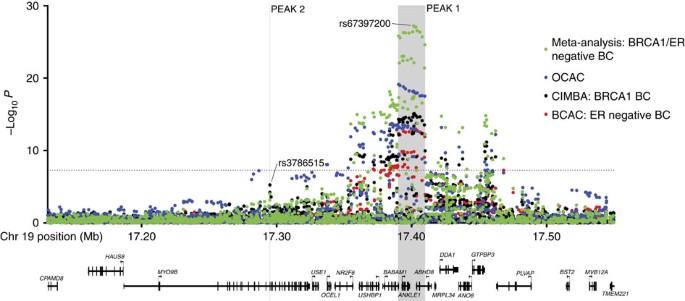Figure 1: Regional association plot disease-specific risk associations. Results for ER negative breast cancer from BCAC, for ovarian cancer from OCAC and forBRCA1mutation carriers with breast cancer from CIMBA are shown. Also shown are the results of a meta-analysis for BRCA1 and general population ER negative breast cancer cases. The grey bars indicate the boundaries of the two association peaks, and the dotted horizontal line indicates the cutoff for genome-wide significance (χ2-testP=5 × 10−8). Previously identified GWAS SNPs are indicated with italic font. Genes in the region are displayed beneath the association results. Genetic association analyses with breast and OC risks A total of 438 SNPs spanning 420 kb at the chromosome 19p13 locus (nucleotides 17,130,000–17,550,000 (NCBI build 37)) were genotyped successfully in the following populations: 46,451 BC cases (of which 7,435 cases had ER-negative tumours) and 42,599 controls from the Breast Cancer Association Consortium (BCAC); 15,438 cases of EOC (of which 9,630 were of serous histology) and 30,845 controls from the Ovarian Cancer Association Consortium (OCAC); and 15,252 BRCA1 mutation carriers from the Consortium of Investigators of Modifiers of BRCA1/2 (CIMBA; 7,797 with BC and 7,455 unaffected; Supplementary Table 1 ). Genotypes for variants identified through the 1,000 genomes project (minor allele frequency (MAF)>0.1%) were imputed for all participants of European ancestry. A total of 2,269 genotyped and imputed SNPs were analysed for their associations with ER-negative BC risk in the general population, 2,311 SNPs with BC/OC risk for BRCA1 mutation carriers, and 2,565 SNPs with risk of serous OC. Results for all SNPs associated with these phenotypes at P <10 −4 are illustrated in Fig. 1 and Supplementary Fig. 1 . Two perfectly correlated SNPs rs61494113 and rs67397200 located between the ANKLE1 and ABHD8 genes demonstrated the strongest association with BC risk among BRCA1 mutation carriers ( χ 2 -test P =7.8 × 10 −16 ) and ER-negative BC in BCAC ( χ 2 -test P =1.3 × 10 −13 , P -meta-analysis=7.3 × 10 −28 ). There was no association for ER-positive BC ( χ 2 -test P =0.21 for rs61494113). The strongest association with invasive and serous OC was for rs4808075 (correlated with rs61494113 with r 2 =0.99) located in the BABAM1 gene ( χ 2 -test P =9.2 × 10 −20 ). 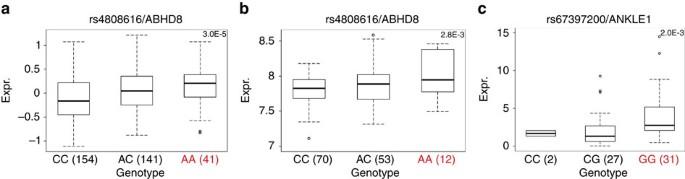Figure 2: Expression quantitative trait locus analyses. Significant eQTL associations identified between rs4808616 andABHD8expression in (a) ovarian cancer tissues and (b) in normal breast tissues. (c) A significant association was also identified between rs4808616 andANKLE1expression in primary normal ovarian/fallopian tube epithelial cell cultures. The horizontal line indicates the median expression, the limits of the boxes denote the first and third quartiles, and the whiskers represent 1.5 times the interquartile range of the data. Outliers are indicated with circles. We observed no associations with risk of other histological subtypes of invasive OC ( Supplementary Table 2 ). 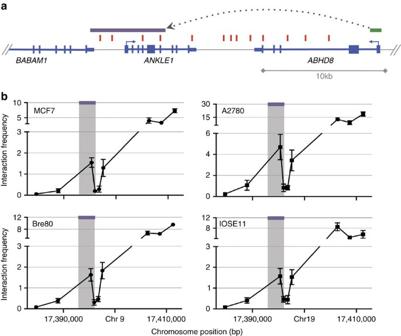Figure 3: Chromosome conformation capture analysis of long-range interactions at the 19p13 region. 3C interaction profiles in breast and ovarian cell lines. 3C libraries were generated withNcoI, with the anchor point set at theABHD8promoter region. (a) A physical map of the region interrogated by 3C is shown, with annotated genes shown in blue, the 13 risk-associated SNPs shown in red, theABHD8promoter fragment shown in green and the position of the interactingNcoI fragment represented by the purple bar (not to scale). (b) Relative interaction frequencies between theABHD8promoter and regions spanning risk associated SNPs in normal breast (Bre80) and ovarian (IOSE11) epithelial cells lines, and in breast (MCF7) and ovarian (A2780) cancer cell lines. A peak of interaction with theABHD8was observed for one region (purple bar) in all four cell lines. There were no interactions detected between the purple region and theBABAM or USHBP1promoters. The interacting region contains four candidate causal SNPs (from left to right) rs4808075, rs10419397, rs56069439 and rs4808076. Error bars represent s.d. (N=3). The correlations between the SNP exhibiting the strongest risk association (rs67397200) in the meta-analysis of BC risk for BRCA1 mutation carriers and ER-negative BC, with the previously reported risk-associated SNPs for breast, OC and BRCA1 -associated BCs can be found in Supplementary Table 3 . Figure 1: Regional association plot disease-specific risk associations. Results for ER negative breast cancer from BCAC, for ovarian cancer from OCAC and for BRCA1 mutation carriers with breast cancer from CIMBA are shown. Also shown are the results of a meta-analysis for BRCA1 and general population ER negative breast cancer cases. The grey bars indicate the boundaries of the two association peaks, and the dotted horizontal line indicates the cutoff for genome-wide significance ( χ 2 -test P =5 × 10 −8 ). Previously identified GWAS SNPs are indicated with italic font. Genes in the region are displayed beneath the association results. Full size image All SNPs with an association P value<0.001 with each phenotype were included in forward stepwise Cox regression models for risks of BRCA1 BC, and logistic regression models for ER-negative BC and serous OC. The most parsimonious models for ER-negative BC and serous OC each included one SNP, rs67397200 for ER-negative BC and rs4808075 for serous OC (referred to as Peak 1). The most parsimonious model in the analysis of BC risk for BRCA1 mutation carriers included two virtually uncorrelated SNPs (pairwise correlation r 2 =0.018) rs61494113 ( P value=4.4 × 10 −16 in conditional regression analysis), and rs3786515 (Peak 2, conditional regression P value=9.6 × 10 −5 , pairwise correlation r 2 =0.018; Fig. 1 ). No other SNP was retained in the model at the P value threshold of 0.0001. Candidate causal variants Peak 1 includes SNPs that encompass the BABAM1, ABHD8 and ANKLE1 gene and are associated with serous OC, ER-negative BC and BC risk for BRCA1 mutation carriers ( Fig. 1 and Supplementary Fig. 1 ); Peak 2 includes SNPs located in the MYO9B gene associated only with BC risk in BRCA1 mutation carriers. SNPs in Peaks 1 and 2 are virtually uncorrelated. To identify the strongest candidate causal SNPs, we computed likelihood ratios of each SNP relative to the SNP with the strongest association in each peak for risks of each phenotype. Due to the similarities in associations between ER-negative BC and BRCA1- associated BC in Peak 1, we computed the likelihood ratios on the basis of the meta-analysis results. Table 1 includes the SNPs that cannot be excluded at a likelihood ratio of >1:100 fold. In Peak 1, all but 12 SNPs can be excluded from being causal for ER-negative BC and BRCA1- associated BC. An additional SNP (rs10424198) cannot be excluded from being causal for serous OC. All 13 SNPs were highly correlated ( r 2 >0.95) and spanned a region of 19.4 kb. In Peak 2, the likelihood ratios of each SNP were calculated on the basis of the BRCA1 association analysis conditional on the top SNP rs61494113. All but seven SNPs correlated with rs3786515 ( r 2 >0.10) cannot be excluded from being the causal SNP for BRCA1- associated BC risk. With the exception of rs3786514 (pairwise r 2 with rs3786515=0.87) all other SNPs had r 2 with rs3786515 between 0.13 and 0.20. Table 1 SNPs associated with risk ovarian cancer, ER-negative breast cancer or breast cancer in BRCA1 carriers at the 19p13 locus. Full size table Associations for BRCA1 and BRCA2 mutation carriers SNPs in Peak 1 were only associated with risk of ER-negative BC for BRCA1 mutation carriers and provided no evidence of association with ER-positive BC for BRCA1 . SNPs in Peak 1 were also associated with OC risk for BRCA1 mutation carriers. 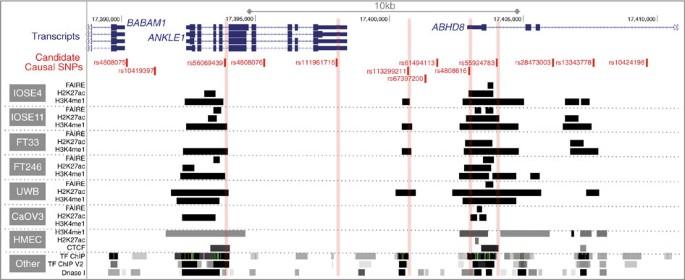Figure 4: Epigenetic marks intersecting candidate causal SNPs in the 19p13 susceptibility region and analyses of UTR SNPs. The thirteen candidate SNPs were aligned with open chromatin and enhancer marks (H3K27ac and H3K4me1) in high-grade serous ovarian cancer cells (UWB1.289 and CaOV3) and ovarian cancer precursor cells (ovarian epithelial cells, IOSE and fallopian epithelial cells, FT). Enhancer and insulator (CTCF) data for human mammary epithelial cells (HMECs) were obtained from ENCODE. Five SNPs coincide with biofeatures in breast and/or ovarian cells (indicated in red). SNPs in Peak 2 were also primarily associated with BRCA1 -related ER-negative BC but there was no evidence of association with OC risk ( Supplementary Table 4 ). SNPs in peak 1 were not associated with overall risk of BC in BRCA2 carriers (for example, rs67397200 HR for BC=1.00 (95% confidence interval (CI): 0.93–0.89)); however, SNP rs67397200 showed evidence of association with OC for BRCA2 mutation carriers (hazards ratio (HR)=1.18, 95% CI: 1.06–1.36, χ 2 -test P =0.0056). SNPs in peak 2 did not show any evidence of association with breast or OC risk for BRCA2 mutation carriers. Associations with risk among BC subtypes None of the Peak 1 SNPs were associated with risk of ER-positive BC. When analyses were restricted to triple negative BC, the odds ratio (OR) estimates for SNPs in Peak 1 were larger than the corresponding OR estimates for ER-negative disease ( Supplementary Table 4 ). There was no evidence of association with ER-negative and HER2-positive BC risk, with the association restricted only to triple-negative BC (test of difference between triple-negative versus ER-negative/HER2+, P -diff=2.2 × 10 −5 for SNP rs61494113). Analysis in Asian and African ancestry studies None of the SNPs in the fine-mapping region were associated with ER-negative BC in samples of Asian ancestry after adjusting for multiple testing ( P values≥0.0018). However, the risk alleles of the 13 candidate causal SNPs in Peak 1 are uncommon in the Asian population (MAF=0.0079–0.011); hence, the power to detect an association was limited and, due to the wide CIs for the estimated ORs for these SNPs, we cannot rule out that the minor allele of these SNPs in Asian subjects is associated with similar level of risk as in Europeans. In samples of African ancestry only rs4808616 (MAF=0.22) showed evidence of association with risk for overall BC or ER-negative disease (OR for BC=1.19, 95% CI:1.02–1.39, χ 2 -test P =0.03; OR for ER-negative BC=1.59, 95% CI: 1.02–2.49, χ 2 -test P =0.04). Functional characterization of the 19p13.1 region Functional characterization focused on the 13 candidate causal SNPs for ER-negative and BRCA1 -associated BC and serous OC in Peak 1, based on the hypothesis that the functional mechanisms mediated by one or more of these SNPs were the same for these phenotypes. Genotype-gene expression associations We used expression quantitative trait locus (eQTL) analyses to evaluate associations between risk SNPs and the expression of genes in a 1 Mb region spanning rs4808075 in: 135 normal breast tissues [29] , 60 normal ovarian and fallopian tube epithelial cell cultures, 391 ER positive BCs [30] , 59 ER-negative BCs [29] and 340 high-grade serous OCs [30] . We identified significant eQTL associations for ABHD8 expression (linear regression P value range 2 × 10 −3 –7 × 10 −3 ) in normal breast tissues and between rs480816 and ABHD8 expression in OCs (linear regression P =3 × 10 −5 ). In both instances the risk allele was associated with higher ABHD8 expression ( Fig. 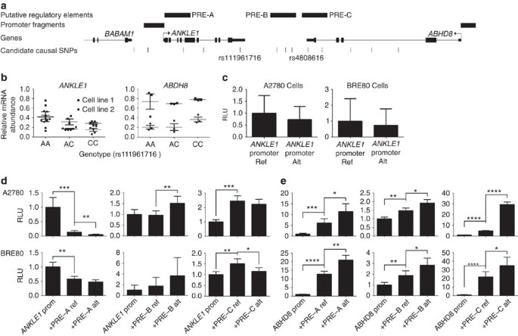Figure 5: Allele specific analysis of susceptibility SNPs. (a) Location of SNPs in putative regulatory elements (PREs) and 5′ untranslated regions. (b) RNA stability assays in primary ovarian epithelial cell lines for risk-associated UTR SNPs inABHD8andANKLE1. Normal ovarian epithelial cell lines carrying different genotypes of the risk SNP rs4808616, located in the 3′ UTR ofABHD8. Rs4808616 is tightly correlated with rs111961716 (R2=0.98) located in the 3′ UTR ofANKLE1. The risk allele of rs111961716 was associated with decreased mRNA stability ofANKLE1compared with the protective allele (P=0.006, ANOVA). Different genotypes of rs4808616 are not associated with the stability theABHD8transcript. (c–e) Luciferase assays to evaluate SNP-dependent promoter and enhancer activity. (c) TheANKLE1promoter SNP did not affectANKLE1expression in ovarian cancer cells (A2780) and normal breast cells (Bre80). (d) Allele-specific activity of PRE-A, PRE-B and PRE-C on theANKLE1promoter. (e) Allele-specific activity of PRE-A, PRE-B and PRE-C onABHD8promoter activity. *P>0.05, **P>0.01, ***P>0.001, ****P>0.0001, two-way ANOVA. RLU, relative light units. 2a , Supplementary Data 1 and 2 and Supplementary Table 5 ). We examined whether risk SNPs were the top eQTL SNPs in this region. rs4808616 was the strongest predictor of ABHD8 expression in OCs. However, in normal breast tissues the top eQTL SNP for ABHD8 was rs11666308 (linear regression P =3.3 × 10 −4 ), a marginally better predictor than rs4808616 (linear regression P =2.8 × 10 −3 ). The two SNPs were correlated ( r 2 =0.79) and regressing out effects of either SNP from the expression levels of ABHD8 and repeating eQTL analysis abolished the eQTL signal for the other SNP, confirming their statistical inseparability. In addition we found significant associations between rs4808616 and NXNL1 expression in OCs (linear regression P =4 × 10 −3 ) and with ANKLE1 expression ( P =0.002) in normal ovarian surface epithelial cells (OSECs). There were no eQTL associations for any other genes in the region. Figure 2: Expression quantitative trait locus analyses. Significant eQTL associations identified between rs4808616 and ABHD8 expression in ( a ) ovarian cancer tissues and ( b ) in normal breast tissues. ( c ) A significant association was also identified between rs4808616 and ANKLE1 expression in primary normal ovarian/fallopian tube epithelial cell cultures. The horizontal line indicates the median expression, the limits of the boxes denote the first and third quartiles, and the whiskers represent 1.5 times the interquartile range of the data. Outliers are indicated with circles. Full size image We also performed allele-specific expression analysis in BC using RNA sequencing data [31] for coding SNPs in ABHD8 (rs56069439) and BABAM1 (rs10424198). Both SNPs were correlated with rs4808616 ( r 2 =0.91). There was a significant association between rs56069439 and the allelic ratio of ABHD8 transcripts (F-test P =0.016) with greater expression associated the risk allele ( Supplementary Fig. 2 ; Supplementary Data 3 ). Chromosome conformation capture Chromosome conformation capture (3C) analysis was used to investigate DNA–DNA interactions between ABHD8 and 5 of 13 candidate causal SNPs in Peak 1. Eight SNPs close to the ABHD8 promoter were too near to be resolved, and the close proximity of candidate causal SNPs to ANKLE1 precluded 3C analysis for this gene. The ABHD8 promoter showed an interaction with a 6.3 kb region ∼ 20 kb telomeric to the gene in both normal breast (Bre80) and ovarian (IOSE11) epithelial cells, and in breast (MCF7) and ovarian (A2780) cancer cell lines ( Fig. 3 ). This region spans the ANKLE1 promoter and includes four candidate causal SNPs: rs4808075, rs10419397, rs56069439 and rs4808076. There was no evidence of interaction for any candidate causal SNP with BABAM1 ( Supplementary Fig. 3 ). Figure 3: Chromosome conformation capture analysis of long-range interactions at the 19p13 region. 3C interaction profiles in breast and ovarian cell lines. 3C libraries were generated with Nco I, with the anchor point set at the ABHD8 promoter region. ( a ) A physical map of the region interrogated by 3C is shown, with annotated genes shown in blue, the 13 risk-associated SNPs shown in red, the ABHD8 promoter fragment shown in green and the position of the interacting Nco I fragment represented by the purple bar (not to scale). ( b ) Relative interaction frequencies between the ABHD8 promoter and regions spanning risk associated SNPs in normal breast (Bre80) and ovarian (IOSE11) epithelial cells lines, and in breast (MCF7) and ovarian (A2780) cancer cell lines. A peak of interaction with the ABHD8 was observed for one region (purple bar) in all four cell lines. There were no interactions detected between the purple region and the BABAM or USHBP1 promoters. The interacting region contains four candidate causal SNPs (from left to right) rs4808075, rs10419397, rs56069439 and rs4808076. Error bars represent s.d. ( N =3). Full size image Annotation of candidate causal SNPs All 13 candidate causal SNPs were located in non-protein coding DNA. We annotated putative functional regulatory elements that coincided with the candidate causal SNPs in normal human mammary epithelial cells (HMECs), and normal fallopian tube and ovarian epithelial cells [19] , and in OC cell lines. Five of the 13 SNPs coincide with regulatory elements that were reproducible in two biological replicate samples ( Fig. 4 ). Three SNPs were located in epigenetic marks in breast and/or ovarian cells: rs55924783 coincided with insulator marks in HMECs and enhancer marks in ovarian cells; rs113299211 coincided with enhancer marks in ovarian cells and is predicted to alter transcription factor binding sites for ELF1, ELK4 and GABP; and rs56069439 coincided with experimentally derived ChIP-seq footprints (for CTCF, ATF2 and ZNF263), enhancer marks in ovarian cells and both enhancer (H3K4me1) and insulator (CTCF) marks in breast cells. Two SNPs were located in 3′-untranslated regions (UTRs) of protein coding genes: rs111961716 in ANKLE1 and rs4808616 in ABHD8 . rs4808616 also coincided with enhancer marks in ovarian and breast cells. Finally, rs10419397 lay within the putative promoter of ANKLE1 , ∼ 1,200 bp from the transcription start site. Figure 4: Epigenetic marks intersecting candidate causal SNPs in the 19p13 susceptibility region and analyses of UTR SNPs. The thirteen candidate SNPs were aligned with open chromatin and enhancer marks (H3K27ac and H3K4me1) in high-grade serous ovarian cancer cells (UWB1.289 and CaOV3) and ovarian cancer precursor cells (ovarian epithelial cells, IOSE and fallopian epithelial cells, FT). Enhancer and insulator (CTCF) data for human mammary epithelial cells (HMECs) were obtained from ENCODE. Five SNPs coincide with biofeatures in breast and/or ovarian cells (indicated in red). Full size image Functional analysis of candidate causal SNPs in UTRs We evaluated the effects on mRNA stability of the SNPs located in 3′ UTRs of ANKLE1 (rs111961716) and ABHD8 (rs4808616, Figs 4 and 5a ) in normal primary ovarian epithelial cell lines carrying different SNP genotypes. RNA transcript abundance was measured after blocking mRNA transcription by treating cells with actinomycin D. For rs111961716, ANKLE1 transcript expression was significantly more stable in cell lines homozygous for the A (risk) allele of rs111961716 compared with heterozygous cells or cells homozygous for the C allele ( P =0.006, analysis of variance; Fig. 5b ). There was no association between ABHD8 mRNA stability and genotypes of rs4808616 ( Fig. 5b ). Figure 5: Allele specific analysis of susceptibility SNPs. ( a ) Location of SNPs in putative regulatory elements (PREs) and 5′ untranslated regions. ( b ) RNA stability assays in primary ovarian epithelial cell lines for risk-associated UTR SNPs in ABHD8 and ANKLE1 . Normal ovarian epithelial cell lines carrying different genotypes of the risk SNP rs4808616, located in the 3′ UTR of ABHD8 . Rs4808616 is tightly correlated with rs111961716 ( R 2 =0.98) located in the 3′ UTR of ANKLE1 . The risk allele of rs111961716 was associated with decreased mRNA stability of ANKLE1 compared with the protective allele ( P =0.006, ANOVA). Different genotypes of rs4808616 are not associated with the stability the ABHD8 transcript. ( c – e ) Luciferase assays to evaluate SNP-dependent promoter and enhancer activity. ( c ) The ANKLE1 promoter SNP did not affect ANKLE1 expression in ovarian cancer cells (A2780) and normal breast cells (Bre80). ( d ) Allele-specific activity of PRE-A, PRE-B and PRE-C on the ANKLE1 promoter. ( e ) Allele-specific activity of PRE-A, PRE-B and PRE-C on ABHD8 promoter activity. * P >0.05, ** P >0.01, *** P >0.001, **** P >0.0001, two-way ANOVA. RLU, relative light units. Full size image Functional analysis of promoter and enhancer SNPs Seven of the 13 candidate causal SNPs in Peak 1 resided either in the ANKLE1 promoter or in putative regulatory elements (PREs-A-C) in breast and ovarian normal and cancer cell lines ( Figs 4 and 5a ). SNP rs10419397 fell within the ANKLE promoter region, but had no effect on promoter activity ( Fig. 5c ). PRE-A contained SNP rs56069439, PRE-B contained SNPs rs113299211, rs67397200, rs61494113 and PRE-C contained SNPs rs4808616 and rs55924783. We examined the effect of these PREs, and of the risk alleles of each SNP cloned into luciferase constructs containing the ABHD8 or ANKLE1 promoters. Inclusion of the reference allele of PREs A, B and C significantly increased ABHD8 promoter activity in both OC (A2780) and normal breast (Bre80) cell lines ( Fig. 5 ). Constructs containing the risk alleles further enhanced ABHD8 promoter activity compared with the reference allele for PREs A, B and C in Bre80 cells ( P values=0.0027, 0.0308 and 0.0342, respectively, two-way analysis of variance (ANOVA)) and for PREs A, B and C in A2780 cells ( P values=0.0193, 0.0115 and <0.0001, respectively, two-way ANOVA; Fig. 5d,e ). Constructs containing the reference allele of PRE-A showed a silencing effect on the ANKLE promoter in both cell types with the risk allele further silencing the activity of the reference allele in A2780 cells ( P =0.0049, two-way ANOVA). The reference allele of PRE-B had no effect on ANKLE promoter activity, while the risk allele significantly increased activity compared with the reference allele in A2780 cells ( P =0.0034, two-way ANOVA). Constructs containing the reference allele of PRE-C significantly increased ANKLE promoter activity in both ovarian ( P =0.0004, two-way ANOVA) and breast cell lines ( P =0.0067, two-way ANOVA). However the risk allele showed a silencing effect on the reference allele in only Bre80 cells ( P =0.0289, two-way ANOVA; Fig. 5d,e ). Functional effects of rs56069439 deletion Collectively, the data above suggested that rs56069439 may regulate the expression of ANKLE1 and/or ABHD8. We used Clustered Regularly Interspaced Short Palindromic Repeats (CRISPR)/Cas9-mediated genome editing to delete a 57 bp region containing the regulatory region that includes rs56069439 in breast (MCF10A) and ovarian (IOSE19) epithelial cells ( Fig. 6a ). Analysis of multiple clones containing confirmed homozygous deletions ( Fig. 6b,c ) indicated a significant reduction in ANKLE1 expression compared with parental cells ( P =0.025, two-tailed paired T -test) and a trend towards reduced ANKLE1 expression in IOSE19 cells ( P =0.29, two-tailed paired T -test; Fig. 6d ). Expression of ABHD8 and BABAM1 was unchanged following deletion of the region containing rs56069439. 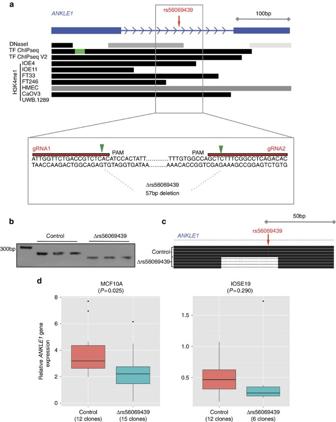Figure 6: Effects of deletion of the putative enhancer containing the rs56069439 risk SNP in breast and ovarian epithelial cells. (a) Illustration of the 57 bp region in an intron ofANKLE1containing rs56069439; H3K4me1 marks overlapped rs56069439 in ovarian, fallopian and breast cells. Location of the two guide RNAs (gRNAs) used to create the stable Δrs56069439 deletion by CRISPR/Cas9 genome editing, cutting sites are indicated with the green arrow. PAM, protospacer adjacent motif. (b) PCR analysis of targeted region in representative MCF10A (breast) epithelial cell clones. Control clones were transfected with the vector backbone only. (c) Verification of deletions by Sanger sequencing, and alignment to the genome using BLAT. (d) Gene expression analysis using TaqMan probes showing downregulation ofANKLE1was associated with deletion of a region containing rs56069439. Figure 6: Effects of deletion of the putative enhancer containing the rs56069439 risk SNP in breast and ovarian epithelial cells. ( a ) Illustration of the 57 bp region in an intron of ANKLE1 containing rs56069439; H3K4me1 marks overlapped rs56069439 in ovarian, fallopian and breast cells. Location of the two guide RNAs (gRNAs) used to create the stable Δrs56069439 deletion by CRISPR/Cas9 genome editing, cutting sites are indicated with the green arrow. PAM, protospacer adjacent motif. ( b ) PCR analysis of targeted region in representative MCF10A (breast) epithelial cell clones. Control clones were transfected with the vector backbone only. ( c ) Verification of deletions by Sanger sequencing, and alignment to the genome using BLAT. ( d ) Gene expression analysis using TaqMan probes showing downregulation of ANKLE1 was associated with deletion of a region containing rs56069439. Full size image In vitro functional analysis of candidate genes We analysed the effects of perturbing ABHD8, ANKLE1 and BABAM1 expression in in vitro models of ‘normal’ breast (MCF10A) and ovarian (IOSE19 (ref. 32 )) epithelial cells. For each gene, we overexpressed full length, green fluorescent protein-tagged constructs, because genes at 19p13 were frequently overexpressed in ovarian and BCs [9] and because eQTL analyses indicated that risk alleles were associated with increased expression of ABHD8 and ANKLE1 . After confirming gene overexpression ( Supplementary Fig. 3a ) we evaluated cell growth, migration and invasion, and anchorage-independent growth ( Fig. 7 and Supplementary Fig. 3b ). Overexpression of ABHD8 caused a significant reduction in cell migration ( P =0.007 in MCF10A; P =0.047 in IOSE19, two-tailed paired T -test) and a decrease in invasion ( P =0.018 in MCF10A; P =0.063 in IOSE19, two-tailed paired T -test; Fig. 7 ). BABAM1 and ANKLE1 overexpression had no effect on these cellular phenotypes for either cell type. 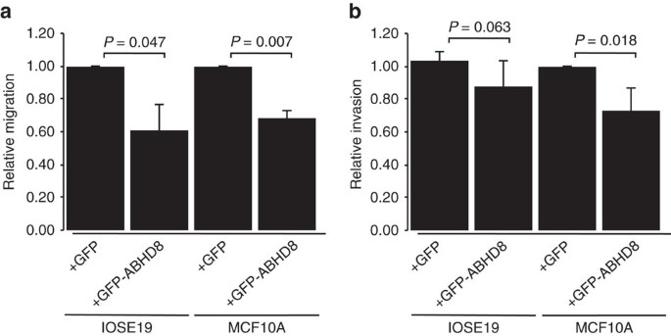Figure 7: Phenotypic effects of overexpressing full lengthABHD8GFP fusion transcript in normal breast and ovarian epithelial cells. (a)ABHD8overexpression induced a significant decrease in migration in both breast (MCF10A) and ovarian (IOSE19) cells; (b)ABHD8overexpression induced a significant decrease in invasion in breast epithelial cells and a similar trend of decreased invasion in ovarian epithelial cells. Figure 7: Phenotypic effects of overexpressing full length ABHD8 GFP fusion transcript in normal breast and ovarian epithelial cells. ( a ) ABHD8 overexpression induced a significant decrease in migration in both breast (MCF10A) and ovarian (IOSE19) cells; ( b ) ABHD8 overexpression induced a significant decrease in invasion in breast epithelial cells and a similar trend of decreased invasion in ovarian epithelial cells. Full size image RNA sequencing was used to profile transcriptomic changes caused by overexpression of ABHD8, ANKLE1 and BABAM1 and pathway analyses performed using Ingenuity Pathway Analysis. We found no indication of significant changes in relevant pathways after overexpressing BABAM1 in breast or ovarian epithelial cells. Cells overexpressing ANKLE1 showed a significant enrichment for cancer-associated and cell growth/proliferation pathways in both breast ( P =3.36 × 10 −6 ) and ovarian ( P =2.43 × 10 −27 ) epithelial cells. Cells overexpressing ABHD8 were enriched for expression changes in cancer related pathways ( P <5.52 × 10 −8 ) and fibrosis pathways ( P <1.23 × 10 −2 , all right-tailed Fisher’s exact tests; Supplementary Tables 6-8 ). Through fine-scale mapping of the 19p13.1 region we have found evidence of two independent regions of genetic association with BC and/or OC risk among women of European ancestry. The minor alleles of all candidate causal variants in Peak 1 conferred increased risks of ER-negative BC and serous OC and increased risks of both cancers for BRCA1 mutation carriers. We were able to rule out associations with ER-positive BC and risks for other OC histotypes. There was weaker evidence that SNPs in Peak 2 were independently associated with BC risk among BRCA1 mutation carriers only. When analyses in BCAC were restricted to triple-negative BC, the strength of association was greater and there was no evidence of association with ER-negative/HER2-positive BC. Thus, our results suggested that these variants are primarily associated with triple-negative BC, the predominant tumour subtype in BRCA1 mutation carriers [33] . These results are in line with previous findings for the initial SNPs identified through GWAS [26] . The increased sample size resulting from combining data from BCAC, OCAC and CIMBA for variants in Peak 1 have enabled us to restrict the likely functional variants at 19p13.1 to 13 SNPs. The 13 candidate causal risk SNPs in this region were the same for both BC and OC leading us to hypothesize that the underlying functional mechanisms are the same in both cancers and the overlap between these SNPs and functional elements provided multiple testable hypotheses, necessitating a range of different functional assays to evaluate their possible causality. Multiple assays were performed in breast and ovarian tissues and cell lines to establish if there is true evidence of pleiotropy. The candidate causal SNPs in Peak 1 clustered around two candidate genes, ANKLE1 and ABHD8 , neither of which have been previously implicated in BC or OC. Proximal to these SNPs is BABAM1 , a gene involved in recruiting BRCA1 to sites of DNA damage [34] , [35] and therefore a compelling candidate gene at this locus. While gene regulation can be mediated across long genomic distances, the majority of interactions occur over a distance of 1 Mb) or less [36] , [37] . We, therefore, evaluated all candidate genes within a 1 Mb region centred on the Peak 1 risk SNPs for eQTL associations. We found significant eQTL associations for ABHD8 in OCs and normal breast tissues, plus allele-specific expression of ABHD8 in BCs, but no compelling evidence for any other gene at this locus. Nonetheless, the identification of ABHD8 as the most likely target susceptibility gene must be treated with some caution as it is plausible that more distant cis -eQTL or even trans -eQTL associations exist for these risk SNPs. Unfortunately, the limited power of eQTL analysis based on the current sample size precluded us from performing genome-wide eQTL analysis to address these hypotheses. The weight of our functional data, in particular the eQTL associations, indicates that ABHD8 is a target of functional SNPs at this locus, and therefore a novel breast and OC susceptibility gene. 3C identified an interaction between a region containing four candidate causal SNPs and the ABHD8 promoter in both breast and OC and normal epithelial cell lines. The luciferase assays of three PREs (including one encompassing rs56069439 in the interacting region) consistently showed that they acted as enhancers, and furthermore the risk-associated alleles of rs56069439, rs113299211, rs67397200, rs61494113, rs4808616 and rs55924783 (within PREs A-C) further increase ABHD8 promoter activity in both breast and ovarian cells. These results were consistent with our eQTL studies and support the hypothesis that increased ABHD8 expression is associated with an increased cancer risk. ABHD8 is a poorly studied lipase [38] . The Achilles heel project identified ABHD8 as a lineage-specific cancer cell vulnerability in OC cell lines [39] and a recent study identified ABHD8 as a potential OC susceptibility gene though its participation in a homeobox transcription factor-centred gene network associated with serous OC risk [40] . Overexpression of ABHD8 led to significant reductions in the invasive and migratory potential of breast and ovarian cells and enriched for genes involved in cellular movement (IOSE19) and mTOR signalling (MCF10A), consistent with the observed changes in invasion and migration. The direction of the effect was opposite to what we might expect from the eQTL data, which might reflect different functions of ABHD8 in different contexts, similar to the observations for another BC susceptibility gene, TOX3 (ref. 41 ). For example, under specific microenvironmental cues or in a tumour cell (rather than the normal cells used in these experiments) increased ABHD8 may promote rather than inhibit migration and invasion. Nonetheless, we cannot unequivocally exclude other genes as the targets of candidate causal variants at this locus, in particular ANKLE1 . The close proximity of the candidate causal SNPs to the ANKLE1 gene precluded 3C analysis; but in the luciferase assays, these same PREs and SNPs had variable, context-dependent effects on ANKLE1 promoter activity. This raises the possibility that the SNPs were cooperatively acting to alter ANKLE1 expression although it was difficult to predict the overall direction of their effects from this assay. We were able to rule out the SNP rs10419397 in the promoter of ANKLE1 as a likely causal variant. The SNP rs111961716 in the 3′-UTR of ANKLE1 was associated with allele-specific ANKLE1 mRNA stability; but stable overexpression of ANKLE1 had no influence on the phenotype of normal breast and ovarian epithelial cells even though pathway after overexpression of ANKLE1 found a significant enrichment for cancer and cell death/proliferation associated pathways in both breast and ovarian epithelial cells. More recently, ANKLE1 has been implicated in DNA damage responses, while other, better-characterized endonucleases (for example, ERCC1) are involved in nucleotide excision repair, which are important for the repair of bulky adducts [42] . This study has highlighted the challenges in establishing causality for both candidate causal SNPs at common variant susceptibility loci and the susceptibility genes targets. The multitude of functional assays that can be used to test allele specific functional activity rarely provide unequivocal evidence of one SNP over another. Genome editing, which allows the creation of isogenic experimental models carrying the different alleles of candidate causal SNP, is emerging as a single assay approach that can evaluate the function of common variants. However, until now the technical challenges of genome editing have restricted its application to two non-coding risk SNPs identified by GWAS at susceptibility loci for prostate cancer and obesity, respectively [22] , [23] . It was beyond the scope of the current study to utilize genome editing to test all 13 candidate causal SNPs in Peak 1 at 19p13 in BC and OC and normal cell line models. Instead, we used CRISPR-Cas9 genome editing to evaluate the effects of a putative enhancer containing most plausible functional SNP (rs56069439) identified from 3C analysis and mapping of putative regulatory elements. This revealed strong functional evidence for a breast/ovarian epithelial cell enhancer, within an intron of ANKLE1 . When this enhancer containing rs56069439 was deleted ANKLE1 expression was significantly reduced, without any reduction in BABAM1 or ABHD8 expression. Further experiments using homology-directed repair will be required to determine if there is allele-specific activity of the rs56069439 SNP in regulating ANKLE1 expression, and to determine whether shadow enhancers are employed to maintain ABHD8 expression [43] . In conclusion, we have performed detailed functional analysis of SNPs and candidate target genes at the 19p13 locus in breast and ovarian normal and cancer cells. ABHD8 is the most likely target gene although we cannot rule out a role for ANKLE1 in the development of breast and OC or the possibility that both genes, acting independently or in synergy may be functional targets of candidate causal SNPs. Using a combination of genetic fine mapping, and a spectrum of in silico and functional assays, seven of thirteen showed evidence of functionality. These data suggest that the underlying functional mechanism(s) at the 19p13 locus may be mediated by many SNPs rather than by a single causal allele. This hypothesis is supported by studies showing tissue-specific enrichment of correlated risk-associated SNPs at susceptibility loci within regulatory biofeatures, including enhancers and transcription factor binding sites [19] , [20] . Such enrichments would not be detected if a single causal SNP at a locus was driving disease development. Taken together these data suggest that common molecular mechanisms are likely to underlie this pleiotropic risk locus. Study populations All specimens used in this study were collected with informed consent and under the approval of local Institutional Review Boards. We used epidemiological and genotype data from studies participating in the BCAC [44] , the OCAC [12] and the CIMBA [45] that have been genotyped using the iCOGS array that included ∼ 200,000 SNPs. BC association consortium Data were available from 52 BC case-control studies, 41 studies of European ancestry, 9 studies of Asian ancestry and 2 studies of African-American ancestry. Details of all studies, the genotyping process and the quality control process have been described elsewhere [6] , [44] , standard sample and genotyping QC criteria were applied. After the quality control process, data on 46,451 cases and 42,599 controls of European ancestry, 6,269 cases and 6,624 controls of Asian ancestry and 1,117 cases and 932 controls of African-American ancestry were available for analysis. Data on the BC ER status were available for 34,509 cases of European ancestry, 7,435 (22%) of whom had ER-negative tumours. OC association consortium Data were available from 41 case-control studies of EOC from OCAC that were genotyped using the iCOGS array [12] . In addition to the OCAC iCOGS data, genotype data were available for stage 1 of three population-based OC genome-wide association studies. The final data set comprised genotype data for 11,069 cases and 21,722 controls from COGS (‘OCAC-iCOGS’), 2,165 cases and 2,564 controls from a GWAS from North America (‘US GWAS’) [46] , 1,762 cases and 6,118 controls from a UK-based GWAS (‘UK GWAS’) [7] , and 441 cases and 441 controls from the Mayo Clinic. All subjects included in this analysis provided written informed consent as well as data and blood samples under ethically approved protocols. Overall, 43 studies from 11 countries provided data on 15,437 women diagnosed with invasive EOC, 9,627 of whom were diagnosed with serous EOC and 30,845 controls from the general population. Consortium of investigators of modifiers of BRCA1/2 Data on BRCA1 mutation carriers were obtained through CIMBA. Eligibility in CIMBA is restricted to females 18 years or older with pathogenic mutations in BRCA1 or BRCA2 . The majority of the participants were sampled through cancer genetics clinics [47] , including some related participants. Fifty-one studies from 25 countries contributed data on BRCA1 mutation carriers who were genotyped using the iCOGS array [45] . After quality control of the phenotypes and genotypes, data were available on 15,252 BRCA1 mutation carriers of whom 7,455 had been diagnosed with BC, 2,639 with ER-negative BC and 1,724 with OC, all of European ancestry. Analyses in BRCA1 mutation carriers focused on assessing associations with BC risk, following the evidence from the original GWAS in BRCA1 mutation carriers [48] . URLs: 1000 Genomes Project, http://www.1000genomes.org/ ; BCAC, http://ccge.medschl.cam.ac.uk/consortia/bcac/index.html ; CIMBA, http://ccge.medschl.cam.ac.uk/consortia/cimba/index.html ; COGS, http://www.cogseu.org/ ; iCOGS, http://ccge.medschl.cam.ac.uk/research/consortia/ icogs/; SNAP https://www.broadinstitute.org/mpg/snap/ ; TCGA, https://tcga-data.nci.nih.gov ; CGHub, https://cghub.ucsc.edu/ iCOGS SNP selection for fine mapping and imputation The fine mapping region was defined as Chromosome 19 positions: 17,130,000–17,550,000 (NCBI build 37). To identify the set of variants potentially responsible for the original GWAS reports, we considered all variants with minor allele frequencies of >0.02 from the 1,000 Genomes Project (March 2010 version) and selected all SNPs correlated ( r 2 >0.1) with either of the two SNPs that had been identified through the BRCA1 and EOC GWAS studies (rs8170 and rs2363956) [12] , [45] , plus an additional set of SNPs that tagged all remaining SNPs in the region with r 2 >0.9. A total of 438 SNPs that were included on iCOGS in the 19p13 region passed QC and were available for the analyses. Data on these SNPs were used to impute the genotypes of all known variants from the 1,000 genomes project (V3, April 2012 release49) using the IMPUTE (version 2) software. After excluding SNPs with MAF<0.001 and SNPs with imputation r 2 accuracy score of ≤0.3, there were 2,269 imputed SNPs in BCAC, 2,565 in OCAC and 2,311 in BRCA1 mutation. BCAC and OCAC association analysis and logistic regression To evaluate the association of each SNP with breast and EOC risk in BCAC and OCAC we used a Wald test statistic based on logistic regression, by estimating the per-allele OR and its s.e. Analyses restricted to specific tumour subtypes (ER-negative BC or high-grade serous EOC) were assessed separately using all available controls. All analyses were adjusted for principal components, described in more detail elsewhere [12] , [44] . Conditional logistic regression was used to assess the evidence that there are multiple independent association signals in the region, by evaluating the associations of genetic variants in the region while adjusting for the SNP with the smallest P value. We considered only SNPs with P values of association of <10 −3 and MAF>0.1% and the most parsimonious model was identified using step-wise forward logistic regression and a threshold of P <10 −4 for retaining SNPs in the model. CIMBA retrospective cohort analysis All associations between genotypes and BC risk in BRCA1 mutation carriers were evaluated using a 1 df per allele trend-test ( P -trend), based on modelling the retrospective likelihood of the observed genotypes conditional on BC phenotypes [49] . To allow for the non-independence among related individuals, an adjusted test statistic was used which took into account the correlation in genotypes [48] . Per allele HR estimates were obtained by maximizing the retrospective likelihood. All analyses were stratified by country of residence. To identify the most parsimonious model that includes multiple SNPs, forward-selection Cox-regression analysis was performed, using the same P value thresholds as in the BCAC and OCAC analysis. This approach provides valid tests of association, although the parameter estimates can be biased [49] , [50] . Parameter estimates for the most parsimonious model were obtained using the retrospective likelihood approach. Meta-analysis It is well established that the majority of BCs in BRCA1 mutation carriers are ER-negative [51] , [52] . To increase the statistical power for identifying the most likely causal variants, we also performed a meta-analysis of the associations of BC risk for BRCA1 mutation carriers and ER-negative BC in the general population (in BCAC) for both genotyped and imputed SNPs. We used an inverse variance approach assuming mixed effects, by combining the logarithm of the per-allele HR for the association with BC risk for BRCA1 mutation carriers and the logarithm of the OR estimate for the association with ER-negative BC in BCAC. eQTL and allele-specific expression analyses Germline genotype data were obtained from the Affymetrix SNP 6.0 (METABRIC) and Illumina 1M-Duo (TCGA HGSOC). No SNPs from Peak 1 and 2 were present on the Affymetrix platform so these genotypes were imputed into the 1000 Genomes European reference panel (March 2012, version 3) using IMPUTE version 2 (ref. 53 ). All analyses were restricted to patients of >90% European ancestry as per LAMP estimates [54] and SNPs with info score >0.3. For METABRIC, gene expression data consisted of probe-level measurements from the Illumina HT-12 v3 microarray platform for a total of 135 samples obtained from normal breast tissue adjacent to tumour and 59 samples obtained from ER-negative breast tumours were analysed. For TCGA HGSOC, gene expression data consisted of measurements from the Agilent 244 K microarray for 340 HGSOC tumours downloaded from the cBioportal. Only genes and probes <1 Mb from the top Peak 1 SNP were analysed. Tumour gene expression data was first adjusted for copy number (TCGA and METBRIC, Affymetrix SNP 6.0 calls) and methylation (TCGA only, Illumina 27 K beta values) using the method of Li et al [31] . Expression QTL analysis was conducted by linear regression with genotypes as predictors, as implemented in the R package Matrix eQTL [55] . Sixty early passage primary normal OSECs and fallopian tube epithelial cells were collected and cultured as previously described [27] , [56] . Briefly, OSECs were harvested from ovaries using a sterile cytobrush and cultured in Medium 199 and MCDB105, mixed in a 1:1 ratio and supplemented with 15% fetal bovine serum (FBS, Hyclone), 10 ng ml −1 epidermal growth factor, 0.5 mg ml −1 hydrocortisone, 5 mg ml −1 insulin (all Sigma, St Louis, MO, USA) and 34 mg protein per ml bovine pituitary extract (Life Technologies). Fresh fallopian specimens were subjected to 48–72 h Pronase (Roche) and DNase I digests to release the epithelial cells. Epithelial cells were pelleted and cultured on collagen in DMEM/F12 supplemented with 10% FBS (Seradigm). RNA was isolated from cell cultures harvested at ∼ 80% confluency using the QIAgen miRNAeasy kit with on-column DNase 1 digestion. 500 ng of RNA was reverse transcribed using SuperScript III First-Strand Synthesis System (Invitrogen). The cDNA was diluted to 10 ng μl −1 and 12.5 ng was used in target specific amplification before real-time PCR using TaqMan PreAmp Master Mix Kit (Applied Biosystems) following Fluidigm’s Specific Target Amplification Protocol. 1.25 μl of the 25 μl pre-amplified cDNA was added to each chip. Each sample was run in triplicate and each experiment included no template controls and no template controls from the cDNA reactions. 96.96 Dynamic Array Integrated Fluidic Circuits (Fluidigm) were loaded with 96 pre-amplified cDNA samples and 96 TaqMan gene expression probes (Applied Biosystems) using the BioMark HD System (Fluidigm). Expression levels for each gene were normalized to the average expression of control genes ( GAPDH and ACTB ). Relative expression levels were calculated using the ΔΔCt method. Correlations between genotype and gene expression were calculated in R 2.14.1. Genotype specific gene expression was compared using the Jonckheere–Terpstra test. Genes with significant eQTL results were validated by individual Taqman (Applied Biosystems, Warrington UK) reactions run on ABI 7900HT Sequence Detection System equipment and analysed with SDS software according to the manufacturer’s instructions. Normal cell line DNAs were analysed on iCOGS arrays to obtain genotype information. We analysed all protein-coding genes within a 1 Mb region of the risk association. The method for allele specific expression analysis has been described previously [31] . Breast and ovarian normal and cancer cell lines Breast and OC cell lines MCF7 (ER+, breast; ATCC #HTB-22) and A2780 (ER+, ovarian; kindly provided by Thomas Hamilton, NCI, Maryland) were grown in RPMI medium with 10% FBS and antibiotics. The normal breast epithelial cell lines Bre-80 (kindly provided by Roger Reddel, CMRI, Sydney) and MCF10A (ATCC #CRL-10317) were grown in DMEM/F12 medium with 5% horse serum, 10 mg ml −1 insulin, 0.5 mg ml −1 hydrocortisone, 20 ng ml −1 epidermal growth factor, 100 ng ml −1 cholera toxin and antibiotics. The phenotypically normal TERT immortalized ovarian epithelial cell lines IOSE11 and IOSE19 (ref. 32 ) were grown in NOSE-CM. All cell lines were maintained under standard conditions, were routinely tested for Mycoplasma and were profiled with short tandem repeats to confirm their identity. Functional annotation of risk SNPs FAIRE-seq and ChIP-seq for H3K27ac and H3K4me1 marks in normal ovarian (IOSE4, IOSE11) and fallopian epithelial cell lines (FT33, FT246) and OC cell lines (CaOV3, UWB1.289) were generated in-house using standard protocols and have been previously described [19] , [27] . Epigenetic marks in HMECs were downloaded from ENCODE (genome.ucsc.edu). Chromosome conformation capture 3C libraries were generated using Nco I as described previously [14] . To quantify interactions by real-time quantitative PCR (qPCR) was performed using primers listed in Supplementary Table 9 . All qPCRs were performed on a RotorGene 6,000 using MyTaq HS DNA polymerase with the addition of 5 mM of Syto9, annealing temperature of 66 °C and extension of 30 s. Each experiments was performed three times in duplicate. The BAC clone (CTD-2278I10) covering the 19p13 region was used to normalize for PCR efficiency and a by reference region within GAPDH used to calculate relative interaction frequencies. All qPCR products were resolved on 2% agarose gels, gel purified and sequenced to verify the 3C product. RNA stability assays For each genotype (two homozygotes and the heterozygote) two early passage primary normal ovarian epithelial cell lines were incubated with actinomycin D for 20 h. RNA was extracted using the QIAgen RNeasy extraction kit and reverse transcribed using MMLV RT enzyme and random hexamers (Promega). Quantitative PCR was performed using TaqMan gene expression probes for ABHD8 (Hs00225984_m1) and ANKLE1 (Hs01094673_g1). Signal for each gene of interest was normalized to signal for ACTB (Hs01060665_g1) and GAPDH (Hs02758991_g1) and relative gene expression calculated using the ΔΔCt method, relative to untreated cells. 18s rRNA (Hs99999901_s1) and MYC (Hs00153408_m1) mRNA levels were included as internal controls. Promoter and allele specific enhancer assays A 1119, bp fragment containing the ABHD8 promoter was cloned into the pGL3 basic luciferase reporter. Reference and risk associated ANKLE1 promoter fragments were synthesized by GenScript and cloned into pGL3 basic. We generated PCR fragments corresponding to PRE A and PRE B and had PRE C haplotype fragments synthesized by GenScript and these were also sub-cloned into ABHD8 and ANKLE1 promoter constructs. PCR primers are listed in Supplementary Table 10 . Bre80 and A2780 cells were transiently transfected with equimolar amounts of luciferase reporter constructs using Renilla luciferase as an internal control reporter. Luciferase was measured 24 h after transfection using Dual-Glo Luciferase (Promega). To correct for any differences in transfection efficiency or cell lysate preparation, Firefly luciferase activity was normalized to Renilla luciferase, and the activity of each construct was measured relative to the promoter alone construct, which had a defined activity of 1. Association was assessed by log transforming the data and performing two-way ANOVA, followed by Dunnett’s multiple comparisons test; for ease of interpretation, values were back transformed to the original scale for the graphs. Genome editing Guide RNAs targeting the region flanking rs56069439 (5′-GTGAGACGGTCAGAACCAAT-3′ and 5′-GTGTCTGAGGCCGAAAGAGC-3′) were designed using the CRISPR design tool from the Zhang lab ( www.crispr.mit.edu ) [57] . The gRNAs were cloned into the lentiCRISPR (Addgene Plasmid 49535) vector by using the BsmBI restriction enzyme site and lentiviral supernatants made by cotransfection of HEK293T cells. IOSE19 and MCF10A cells were transduced with viral supernatants and infected cells selected using 400 ng ml −1 and 500 ng ml −1 puromycin (Sigma Aldrich) respectively. Selected cells were sorted into single cells using flow cytometry and expanded in vitro. Screening for clones containing the deletion was performed using the following primers: Forwards: 5′-CCCTGACATCCAGGGTCTTC-3′ and Reverse: 5′-AGTCCAGCGTCTCATCGGTA-3′. For sequence verification of the deletion the following primers were used: Forwards: 5′-TTCTGGACCAGTCCCTGACA-3′ and Reverse: 5′-CAGCGTCTCATCGGTAGGTC-3′. RNA was isolated from positive clones using the Zymo Quick-RNA kit and reverse transcribed using Superscript III (Life Technologies). Real time gene expression analysis was performed using TaqMan probes, as described above. In vitro analysis of candidate genes The three candidate genes were overexpressed as green fluorescent protein fusion proteins. The BABAM1 overexpression construct was a kind gift from Dr S Elledge [58] . ANKLE1 and ABHD8 contructs were purchased from Genecopoeia. Virus was made in-house by cotransfection of HEK293Ts and used to transduce MCF10A and IOSE19 cells. Positive cells were selected using 400 ng ml −1 (for IOSE19 cells) or 500 ng ml −1 (for MCF10A cells) puromycin. Anchorage dependent and independent growth assays were performed as previously described [32] , [59] . For invasion and migration assays Millipore luminescent transwell assays (24 well plate format) were used, following the manufacturer’s protocol. Data availability The relevant SNP genotype data underpinning these analyses can be accessed by applying to the OCAC, BCAC and CIMBA consortia (see URLs). EQTL data are available in supplementary information . All other data are available on request. How to cite this article: Lawrenson, K. et al . Functional mechanisms underlying pleiotropic risk alleles at the 19p13.1 breast-ovarian cancer susceptibility locus. Nat. Commun. 7:12675 doi: 10.1038/ncomms12675 (2016).